Adaptive mutations in NEP compensate for defective H5N1 RNA replication in cultured human cells Infection of mammals by avian influenza viruses requires adaptive mutations to achieve high-level replication in the new host. However, the basic mechanism underlying this adaptation process is still unknown. Here we show that avian polymerases, lacking the human signature PB2-E627K, are incapable of generating usable complementary RNA templates in cultured human cells and therefore require adaptation. Characterization of the highly pathogenic human H5N1 isolate A/Thailand/1(KAN-1)/2004 that retained the avian PB2-E627 reveals that the defect in RNA replication is only partially compensated by mutations in the polymerase. Instead, mutations in the nuclear export protein are required for efficient polymerase activity. We demonstrate that adaptive mutations in nuclear export proteins of several human isolates enhance the polymerase activity of avian polymerases in human cultured cells. In conclusion, when crossing the species barrier, avian influenza viruses acquire adaptive mutations in nuclear export protein to escape restricted viral genome replication in mammalian cells. To cross the species barrier to mammals, avian influenza viruses depend on the acquisition of adaptive mutations that allow efficient viral replication in the new host. Besides amino-acid changes in the hemagglutinin and NS1 proteins [1] , [2] , [3] , mutations in the viral polymerase proteins have been shown to be major determinants of adaptation [2] , [4] , [5] . Whereas avian influenza A virus isolates almost exclusively contain glutamic acid at position 627 in the polymerase PB2 protein (PB2-E627), this position is frequently mutated to lysine in human-derived isolates (PB2-E627K), including H5N1 isolates that cause a high morbidity in humans. The PB2-E627K mutation was shown to increase viral polymerase activity in mammalian cells [2] , [6] and is accompanied by improved viral replication at low temperatures [6] , [7] . Furthermore, enhanced binding of the viral polymerase to the nucleoprotein (NP) in human cells [8] has been discussed as a consequence of this mutation. Intriguingly, fatal viral infections of humans with avian viruses of the H5N1 subtype that have retained the avian like PB2-E627 have been reported [9] . Moreover, the 2009 H1N1 pandemic virus also harbours PB2-E627, but additionally possesses a lysine at position 591 (PB2-E591K), which is able to partially, but not completely, compensate for the lack of the PB2-E627K mutation [10] , [11] , suggesting that other adaptive factors may account for the efficient replication of these viruses in humans. Other mutations in PB2, known to have a role in host adaptation, are the exchange of aspartic acid with asparagine at position 701 (PB2-D701N), which can confer high pathogenicity to avian H5N1 and H7N7 viruses in mice [4] , [12] and the substitution of threonine with alanine at position 271 (PB2-T271A), which has been suggested to enhance polymerase activity in mammalian cells [13] . Furthermore, adaptation to human importin α might have a crucial role in interspecies transmission and pathogenicity [15] , [16] . The human H5N1 isolate KAN-1 (A/Thailand/1(KAN-1)/2004) [17] , originating from an avian influenza outbreak in Thailand in 2003, also encodes PB2-E627, yet, nonetheless, is highly pathogenic in different animal models, including mice and ferrets [14] , [15] . To understand the molecular basis of this pathogenicity, we generated a probable avian precursor virus (AvianPr) of KAN-1, devoid of adaptive mutations. Using AvianPr, we could show that an avian influenza polymerase, containing PB2-E627, exhibits a distinct defect in the replication of the viral genome (vRNA) in mammalian cells in culture. This malfunction in vRNA replication is manifested by the generation of defective complementary ribonucleoprotein complexes (cRNPs), which cannot be utilized as templates for efficient vRNA synthesis. We can show that this defect in vRNA replication is compensated by the PB2-E627K mutation. Furthermore, by introducing the pathogenicity-enhancing mutation M16I of KAN-1 nuclear export protein (NEP) and other mutations found in human H5N1 isolates into the AvianPr NEP, respectively, we can demonstrate that NEP increases the polymerase activity of avian H5N1 viruses that harbour PB2-E627 in human cultured cells. Taken together, our data suggest that the defect of avian H5N1 viruses in vRNA replication in human cells can be either compensated by the PB2-E627K mutation or adaptive mutations in NEP. Identification of pathogenicity determinants of KAN-1 The rapid evolution of H5N1 influenza in birds [16] usually prevents isolation and assignment of a direct avian precursor to pathogenic human viruses. Discrimination between non-adaptive amino-acid changes in avian isolates that have been acquired during circulation in the avian host and adaptive mutations that specifically facilitate infection in humans is a difficult task. To circumvent this problem, we used the influenza Virus Resource Database [17] and compared the amino-acid sequences of various H5N1 viruses of avian or human origin ( Supplementary Table S1 ). Reversion of non-avian-like amino acids in the highly pathogenic human-derived H5N1 strain A/Thailand/1(KAN-1)/2004 (KAN-1) to avian-like residues allowed us to generate the sequence of a probable low-pathogenic AvianPr of KAN-1 that differs in 7 positions in PB2, PB1, PA, NA, NS1 and NEP ( Fig. 1a ). To evaluate the pathogenicity of AvianPr in mammals, recombinant KAN-1 and AvianPr viruses were generated using reverse genetics. Both viruses showed comparable growth kinetics in avian cells in culture ( Fig. 1b ), whereas viral growth of AvianPr was delayed in mammalian MDCK cells compared with KAN-1 ( Fig. 1c ). Similarly, infection of BALB/c mice revealed a strong attenuation of the AvianPr virus, as was demonstrated by an increase in the 50% lethal dose 50 (LD 50 ) of ~3 log 10 compared with the KAN-1 virus ( Fig. 1d ). These results suggest that the identified mutations in KAN-1 indeed contribute to the pathogenicity of this virus in mice. 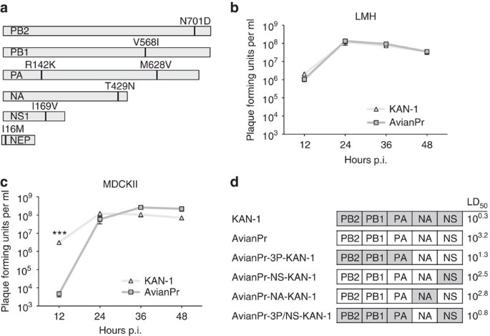Figure 1: Characterization of KAN-1 and AvianPr reassortant viruses in cell culture and mice. (a) Amino-acid differences between indicated viral proteins of KAN-1 and the avian precursor AvianPr. (b,c) Growth curves of infected cell culture. Confluent canine MDCKII (b) and avian LMH (c) cells were infected with an MOI of 0.001 and incubated at 37 °C. At the indicated time points post infection virus titre in the supernatant was analysed by plaque assay. Error bars indicate the standard error of the mean of three independent experiments. Student'st-test was performed to determine thePvalue. ***P<0.001. (d) LD50of KAN-1, AvianPr, and the indicated AvianPr reassortant viruses after intranasal infection of BALB/c mice (n=5 per group). Reassortant viruses include AvianPr harbouring either all three polymerase segments (AvianPr-3P-KAN-1), NS (AvianPr-NS-KAN-1), NA (AvianPr-NA-KAN-1) or both the NS and polymerase segments (AvianPr-3P/NS-KAN-1) of KAN-1. Segments originating from KAN-1 virus are highlighted in grey. Figure 1: Characterization of KAN-1 and AvianPr reassortant viruses in cell culture and mice. ( a ) Amino-acid differences between indicated viral proteins of KAN-1 and the avian precursor AvianPr. ( b , c ) Growth curves of infected cell culture. Confluent canine MDCKII ( b ) and avian LMH ( c ) cells were infected with an MOI of 0.001 and incubated at 37 °C. At the indicated time points post infection virus titre in the supernatant was analysed by plaque assay. Error bars indicate the standard error of the mean of three independent experiments. Student's t -test was performed to determine the P value. *** P <0.001. ( d ) LD 50 of KAN-1, AvianPr, and the indicated AvianPr reassortant viruses after intranasal infection of BALB/c mice ( n =5 per group). Reassortant viruses include AvianPr harbouring either all three polymerase segments (AvianPr-3P-KAN-1), NS (AvianPr-NS-KAN-1), NA (AvianPr-NA-KAN-1) or both the NS and polymerase segments (AvianPr-3P/NS-KAN-1) of KAN-1. Segments originating from KAN-1 virus are highlighted in grey. Full size image To dissect the contribution of the individual mutations in more detail, reassortant viruses of the two strains were generated ( Fig. 1d ). Introduction of the KAN-1 polymerase into the low-pathogenic avian precursor (AvianPr-3P-KAN-1) resulted in reduction of the LD 50 from 10 3.2 to 10 1.3 ( Fig. 1d ), indicating that the mutations in the polymerase proteins are required for the pathogenicity of the KAN-1 virus in mice. However, introduction of the KAN-1 NS (AvianPr-NS-KAN-1) or NA segments (AvianPr-NA-KAN-1) also enhanced the pathogenicity of AvianPr, leading to a decrease in the LD 50 by 0.7 log 10 and 0.4 log 10 , respectively ( Fig. 1d ). Interestingly, AvianPr containing both the KAN-1 polymerase, together with the KAN-1 NS segment (AvianPr-3P/NS-KAN-1), showed high pathogenicity as demonstrated by the low LD 50 of 10 0.8 , suggesting that either NS1 or NEP or both are important cofactors for KAN-1 pathogenicity. Although mice infected with 10 4 plaque-forming units (PFU) of AvianPr succumbed to infection, there was a considerable delay in weight loss ( Fig. 2 ), suggesting the emergence of virus mutants harbouring disease-enhancing adaptive mutations. Interestingly, sequencing of the carboxy terminus of PB2, from infected mouse lung tissue, revealed that all viruses containing the avian polymerase acquired adaptive mutations in PB2 during mouse infection, as well as 63% of the AvianPr-3P-KAN-1 viruses containing the KAN-1 polymerase and 78% of the AvianPr-NS-KAN-1 viruses containing the NS segment of KAN-1 combined with the AvianPr polymerase ( Table 1 ). However, in mice infected with the reassortant virus AvianPr-3P/NS-KAN-1 harbouring the KAN-1 polymerase and NS segment, no adaptive mutations in PB2 appeared, indicating that this virus might be sufficiently adapted to replicate in the mammalian host. 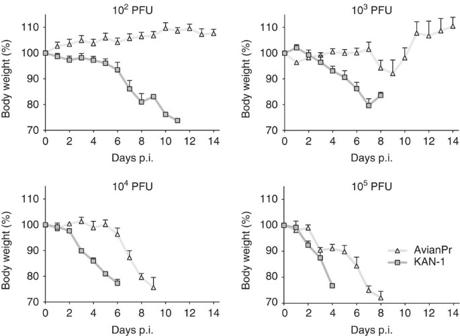Figure 2: Weight curves of infected BALB/c mice. 6–8 weeks old female BALB/c mice (n=5 per group) were infected intranasally with indicated infectious doses of either AvianPr or KAN-1 virus. Weight loss was monitored for 14 days post-infection (p.i.). Error bars indicate the s.e. of the mean. Figure 2: Weight curves of infected BALB/c mice. 6–8 weeks old female BALB/c mice ( n =5 per group) were infected intranasally with indicated infectious doses of either AvianPr or KAN-1 virus. Weight loss was monitored for 14 days post-infection (p.i.). Error bars indicate the s.e. of the mean. Full size image Table 1 Adaptive mutations in mice. Full size table KAN-1 mutations in polymerase partially increase its activity Although introduction of the KAN-1 polymerase increased the pathogenicity of AvianPr in mice, the appearance of compensatory mutations in PB2, during mouse infection, suggests an incomplete adaptation of the KAN-1 polymerase to the mammalian host. We, therefore, compared the polymerase activity of KAN-1 with the human H5N1 isolate A/Viet Nam/1203/2004 (Vn-1203), a highly active prototypical human H5N1 strain that encodes PB2-K627 ( Fig. 3a ), using a polymerase reconstitution assay in human cultured cells. For comparison, we included both the AvianPr and an AvianPr polymerase containing PB2-E627K (AvianPr-PB2-E627K). Measuring reporter gene activity at 3, 6, 9, 12 h post-transfection, we found that the KAN-1 polymerase activity was ~1 log 10 lower compared with the Vn-1203 and AvianPr-PB2-E627K polymerases ( Fig. 3b ). However, after 24 h, all three polymerases reached the same activity, indicating that the KAN-1 polymerase has a functional disadvantage in human cultured cells, but is able to reach high productivity at later time points. As expected, the AvianPr polymerase lacking the adaptive mutations showed the lowest polymerase activity, at least 2 log 10 less than the PB2-E627K containing polymerases at 9, 12 and 24 h post-transfection ( Fig. 3b ). In contrast, all polymerases exhibited comparable activity in avian LMH cells ( Fig. 3c ), thereby confirming the functionality of the AvianPr polymerase, and indicating that the enhancing effect of the adaptive mutations is specific to mammalian, but not avian cells in culture. Detailed analysis of single amino-acid substitutions highlighted the importance of the mutations PB2-D701N and PA-K142R for KAN-1 and PB2-E627K and PA-K142E for Vn-1203 polymerase activity in mammalian ( Fig. 3d–f ), but not avian cells in culture ( Fig. 3g–i ). The increase in polymerase activity observed in human cultured cells additionally correlated with enhanced formation of viral ribonucleoprotein complexes (RNPs) ( Fig. 3j–k ), as previously described [8] . 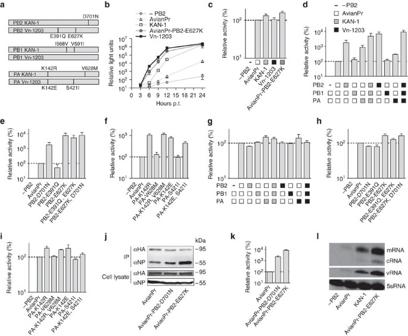Figure 3: Activity of H5N1 polymerases in cell cultures. (a) Cartoon depicting the amino-acid differences between the polymerase subunits PB2, PB1 and PA of the H5N1 isolates KAN-1 and Vn-1203. (b) To determine the polymerase activity of the indicated viruses in a time-dependent manner post-transfection (p.t.), HEK293T cells were transiently transfected with expression plasmids coding for the corresponding PB2, PB1, PA and NP proteins, a human polymerase I-driven vRNA-luciferase reporter plasmid and a renilla-expressing plasmid. Omission of PB2 (−PB2) was used as a negative control. Renilla activity was used to normalize variation in transfection efficiency. Error bars indicate the standard error of the mean of three independent experiments. (c) Relative polymerase activity in avian LMH cells. (d–f) Relative polymerase activity in HEK293 T cells after exchange of the indicated polymerase subunits (d) or mutation of the indicated amino-acid positions in PB2 (e) or PA (f). (g–i) Relative polymerase activity in avian LMH cells after exchange of the indicated polymerase subunits (g) or mutation of the indicated amino-acid positions in PB2 (h) or PA (i). (j,k) RNP formation of reconstituted polymerases in HEK293T. Reconstitution of the AvianPr polymerase complex was carried out, as described in (b), using expression plasmids coding for PB2-HA with the annotated mutation. A cell extract was prepared 24 h post-transfection determining the reporter activity (j) and subjected for co-immunoprecipitation (IP) experiments using anti-HA antibodies. Polymerase activity was normalized to renilla activity, and the levels obtained with the AvianPr-HA-PB2 were set to 100%. Error bars indicate the standard error of the mean of three independent experiments. The viral NP and PB2 were detected by western blot. (l) Determination of the mRNA, cRNA and vRNA levels by primer extension analysis after reconstitution of the AvianPr, KAN-1 and AvianPr-PB2-E627K polymerases 24 h post-transfection, using segment 6. Determination of the 5sRNA levels served as an internal loading control. Figure 3: Activity of H5N1 polymerases in cell cultures. ( a ) Cartoon depicting the amino-acid differences between the polymerase subunits PB2, PB1 and PA of the H5N1 isolates KAN-1 and Vn-1203. ( b ) To determine the polymerase activity of the indicated viruses in a time-dependent manner post-transfection (p.t. ), HEK293T cells were transiently transfected with expression plasmids coding for the corresponding PB2, PB1, PA and NP proteins, a human polymerase I-driven vRNA-luciferase reporter plasmid and a renilla-expressing plasmid. Omission of PB2 (−PB2) was used as a negative control. Renilla activity was used to normalize variation in transfection efficiency. Error bars indicate the standard error of the mean of three independent experiments. ( c ) Relative polymerase activity in avian LMH cells. ( d – f ) Relative polymerase activity in HEK293 T cells after exchange of the indicated polymerase subunits ( d ) or mutation of the indicated amino-acid positions in PB2 ( e ) or PA ( f ). ( g – i ) Relative polymerase activity in avian LMH cells after exchange of the indicated polymerase subunits ( g ) or mutation of the indicated amino-acid positions in PB2 ( h ) or PA ( i ). ( j , k ) RNP formation of reconstituted polymerases in HEK293T. Reconstitution of the AvianPr polymerase complex was carried out, as described in ( b ), using expression plasmids coding for PB2-HA with the annotated mutation. A cell extract was prepared 24 h post-transfection determining the reporter activity ( j ) and subjected for co-immunoprecipitation (IP) experiments using anti-HA antibodies. Polymerase activity was normalized to renilla activity, and the levels obtained with the AvianPr-HA-PB2 were set to 100%. Error bars indicate the standard error of the mean of three independent experiments. The viral NP and PB2 were detected by western blot. ( l ) Determination of the mRNA, cRNA and vRNA levels by primer extension analysis after reconstitution of the AvianPr, KAN-1 and AvianPr-PB2-E627K polymerases 24 h post-transfection, using segment 6. Determination of the 5sRNA levels served as an internal loading control. Full size image Next, we performed a primer extension assay to analyse the accumulation of the three viral RNA species, messenger RNA (mRNA), complementary RNA (cRNA) and genomic RNA (vRNA) produced by the AvianPr, KAN-1 and AvianPr-PB2-E627K polymerases. In agreement with the results from the reporter assay ( Fig. 3b ), the AvianPr polymerase produced very low amounts of vRNA and mRNA and no detectable cRNA ( Fig. 3l ). Interestingly, the KAN-1 polymerase produced higher amounts of vRNA and mRNA than AvianPr, but also only minor amounts of cRNA. In comparison, the highly active AvianPr-PB2-E627K polymerase produced high amounts of all three viral RNA species, correlating with the strong reporter gene activity in the reconstitution assay ( Fig. 3l ). In summary, these results indicate that the adaptive mutations in the KAN-1 polymerase are not able to fully compensate for the lack of PB2-E627K and are insufficient to reach the activity of the PB2-E627K containing polymerases. PB2-E627K compensates for a defect in viral RNA replication According to the primer extension analysis, the AvianPr polymerase, which is identical to several avian isolates ( Supplementary Table S1 ) produces substantially lower amounts of viral cRNA, vRNA and mRNA compared with AvianPr-PB2-E627K polymerase. However, it remains unclear if this impairment is a result of a deficiency in c/vRNA synthesis (replication), mRNA synthesis (transcription), or a combination thereof. To clarify which function of the polymerase is impaired in avian strains, we performed a PB2 complementation assay in human cultured cells using the polymerase reconstitution system. In this assay, we co-expressed a modified AvianPr PB2 subunit (PB2-E627K-Tdef) that harbours both the adaptive mutation E627K as well as mutations in the cap-binding region that diminish the cap-binding activity [18] and therefore leads to inefficient transcription of mRNA from vRNA. If AvianPr is only defective for RNA replication in human cultured cells, the avian precursor polymerase should be able to complement the transcription defect of PB2-E627K-Tdef, whereas no complementation should occur if the AvianPr polymerase also has a defect in transcription ( Fig. 4a ). As shown in Fig. 4b , polymerase containing AvianPr PB2 (PB2-AvianPr) produced only low levels of all three RNA species. In contrast, the transcription-deficient polymerase (PB2-E627K-Tdef) produced high amounts of vRNA and cRNA, but no detectable amounts of mRNA. Co-expression of equal amounts of PB2-AvianPr and PB2-E627K-Tdef polymerases resulted in the restoration of full RNA synthesis and the production of all three RNA species to levels resembling the PB2-E627K phenotype. These results suggest that the AvianPr polymerase is not defective for mRNA synthesis and can synthesize mRNA when the vRNA template is provided in trans. Using the luciferase reporter construct, we could similarly observe strongly reduced reporter gene activity for PB2-AvianPr and PB2-E627K-Tdef, while the activity was restored by co-expression of both polymerases ( Fig. 4c ), confirming the results observed by primer extension analysis. We therefore conclude that the non-adapted AvianPr polymerase does not harbour a defect in viral mRNA synthesis. Supporting this hypothesis, AvianPr and AvianPr-E627K recombinant viruses exhibited equal primary mRNA synthesis after infection of HEK293T cells in the presence of cycloheximide ( Fig. 4d ), conditions that prevent viral RNA replication. 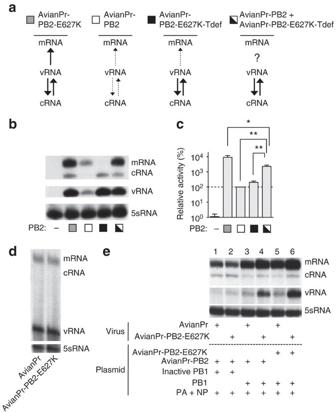Figure 4: Polymerase complementation assay. (a) Cartoon depicting the various PB2 mutants and the expected polymerase activity in the presence of these mutants. AvianPr-PB2-E627K-Tdef represents the AvianPr PB2 harbouring the mutation E627K and two mutations (E361A, F404A) in the cap-binding domain. Black solid arrows refer to synthesis of high RNA levels by the indicated polymerase; arrows with dotted lines indicate synthesis of low vRNA amounts. The question mark indicates unknown levels of RNA synthesis. (b) Determination of the mRNA, cRNA and vRNA levels by primer extension analysis after reconstitution of the AvianPr with the indicated PB2 subunits using specific primers for segment 6. Determination of the 5sRNA levels served as an internal loading control. For reconstitution the total amount of 50 ng of PB2-expressing plasmids were transfected. The complementation assays included 25 ng of AvianPr-PB2 and 25 ng AvianPr-PB2-E627K-Tdef. Omission of PB2 (−PB2) was used as a negative control. (c) Luciferase reporter activities of mutant polymerases 24 h post-transfection after reconstitution of the indicated polymerases in HEK293T cells. For each reconstitution, a total amount of 50 ng of PB2-expressing plasmids were used. The complementation assays included 25 ng of AvianPr-PB2 and 25 ng AvianPr-PB2-E627K-Tdef. Error bars indicate the standard error of the mean of three independent experiments. Student'st-test was performed to determine thePvalue. *P<0.05; **P<0.01. (d) Primary viral transcription in HEK293T cells infected with an MOI of 5 of either AvianPr or AvianPr-PB2-E627K and treated with 100 μg ml−1cycloheximide. Cells were collected 4 h p. i., and mRNA, cRNA and vRNA levels were determined using primer extension analysis with primers specific for segment 6. Levels of cellular 5sRNA served as internal loading control. (e) Rescue of cycloheximide-mediated inhibition of influenza virus replication. Human 293T cells were transiently transfected with the indicated polymerase subunits and viral NP and subsequently infected with the indicated virus strain at an MOI of 5. vRNA species were analysed 6 h post infection by primer extension using specific primer for segment 1. Figure 4: Polymerase complementation assay. ( a ) Cartoon depicting the various PB2 mutants and the expected polymerase activity in the presence of these mutants. AvianPr-PB2-E627K-Tdef represents the AvianPr PB2 harbouring the mutation E627K and two mutations (E361A, F404A) in the cap-binding domain. Black solid arrows refer to synthesis of high RNA levels by the indicated polymerase; arrows with dotted lines indicate synthesis of low vRNA amounts. The question mark indicates unknown levels of RNA synthesis. ( b ) Determination of the mRNA, cRNA and vRNA levels by primer extension analysis after reconstitution of the AvianPr with the indicated PB2 subunits using specific primers for segment 6. Determination of the 5sRNA levels served as an internal loading control. For reconstitution the total amount of 50 ng of PB2-expressing plasmids were transfected. The complementation assays included 25 ng of AvianPr-PB2 and 25 ng AvianPr-PB2-E627K-Tdef. Omission of PB2 (−PB2) was used as a negative control. ( c ) Luciferase reporter activities of mutant polymerases 24 h post-transfection after reconstitution of the indicated polymerases in HEK293T cells. For each reconstitution, a total amount of 50 ng of PB2-expressing plasmids were used. The complementation assays included 25 ng of AvianPr-PB2 and 25 ng AvianPr-PB2-E627K-Tdef. Error bars indicate the standard error of the mean of three independent experiments. Student's t -test was performed to determine the P value. * P <0.05; ** P <0.01. ( d ) Primary viral transcription in HEK293T cells infected with an MOI of 5 of either AvianPr or AvianPr-PB2-E627K and treated with 100 μg ml −1 cycloheximide. Cells were collected 4 h p. i., and mRNA, cRNA and vRNA levels were determined using primer extension analysis with primers specific for segment 6. Levels of cellular 5sRNA served as internal loading control. ( e ) Rescue of cycloheximide-mediated inhibition of influenza virus replication. Human 293T cells were transiently transfected with the indicated polymerase subunits and viral NP and subsequently infected with the indicated virus strain at an MOI of 5. vRNA species were analysed 6 h post infection by primer extension using specific primer for segment 1. Full size image We then investigated whether the replication defect of AvianPr is caused by impairment in cRNA synthesis, as no cRNA production by AvianPr was detectable in the primer extension assay ( Fig. 4d ). Because this could be caused by impaired cRNA synthesis and/or rapid degradation of synthesized cRNA, we performed a cRNA stabilization assay [19] . As described by others, cRNA synthesis can be observed by pre-expression of NP and a catalytically inactive polymerase, containing an inactive PB1 subunit [19] before viral infection in the presence of cycloheximide [19] . As shown in Fig. 4e (lane 1 and 2), in AvianPr- and AvianPr-E627K-infected human cells in culture, both polymerases produce substantial and equivalent amounts of cRNA. To further determine whether the cRNA transcripts can be utilized as templates for vRNA synthesis, we overexpressed functional AvianPr or AvianPr-PB2-E627K polymerase subunits and NP before infection and cycloheximide-treatment. Intriguingly, in human cultured cells infected with AvianPr, both polymerases failed to produce vRNA ( Fig. 4e , lanes 3 and 5) but synthesized substantial amounts of vRNA in AvianPr-PB2-E627K-infected cells ( Fig. 4e , lanes 4 and 6). Thus, avian polymerases lacking PB2-E627K appear incapable of providing bona fide cRNA templates in human cultured cells (Discussion). These data suggest a general requirement of avian influenza polymerases to increase their RNA replication efficiency in mammalian cells, which can be achieved by the adaptive mutation E627K in PB2. On the basis of the observation that the KAN-1 polymerase is not fully adapted to mammalian cells in culture, we speculated that an additional cofactor is necessary for efficient RNA replication by KAN-1. The NEP protein of KAN-1 is involved in host adaptation As we could show that the NS segment contributes to viral pathogenicity of KAN-1, we speculated that either NS1 or NEP, both encoded by this segment, could have a stimulatory effect on viral polymerase activity in human cultured cells. Because of overlapping open reading frames of the two proteins, the single mutation in the NS segment of the KAN-1 virus results in an amino-acid change at position 174 (valine to isoleucine) in the NS1 protein, and at position 16 (methionine to isoleucine) in NEP ( Fig. 5a ). To elucidate whether these amino-acid changes in NS1 or NEP stimulate the activity of a polymerase lacking adaptive mutations, we determined the polymerase activity of AvianPr in the presence of either protein in human cultured cells. Co-transfection of either KAN-1 or AvianPr NS1 expression plasmids resulted in a reduction of AvianPr reporter activity ( Fig. 5b ), suggesting that the mutation in KAN-1 NS1 is not important for viral polymerase function. In contrast, we could observe an enhancement of the AvianPr reporter activity by the NEP proteins of both the AvianPr and KAN-1 virus at low plasmid concentrations ( Fig. 5c ). However, reporter gene activity was up to 51-fold higher on co-expression of the KAN-1 NEP compared with NEP of AvianPr. This indicates that the mutation M16I in the KAN-1 NEP leads to an enhancement of the polymerase stimulating property of the avian NEP ( Fig. 5c ). On the other hand, we observed an inhibition of reporter gene activity at high plasmid concentrations for both NEP proteins. This inhibitory effect was much more pronounced for the AvianPr NEP on co-transfection, leading to a reduction of reporter gene activity to background levels ( Fig. 5c ). Expression levels of the AvianPr and KAN-1 NEP in human HEK293T cells were comparable ( Fig. 7c ). At low levels of transfected NEP expression plasmids, primer extension analysis revealed that AvianPr NEP slightly increased the level of cRNA but not mRNA ( Fig. 5d ). In contrast, KAN-1 NEP greatly enhanced the synthesis of all viral RNA species, including cRNA. At tenfold higher amounts of transfected NEP-expression plasmids, viral polymerase was inhibited by NEP of both KAN-1 and AvianPr; however, the inhibitory effect of KAN-1 NEP was less pronounced. Next, we tested whether the stimulatory effect of KAN-1 NEP is able to compensate the inefficient adaptation of the KAN-1 polymerase in a polymerase reconstitution assay, as observed in Fig. 3b . Co-expression of KAN-1 polymerase with KAN-1 NEP resulted in similar reporter activity as AvianPr-PB2-E627K co-expressed with AvianPr-NEP ( Fig. 5e ). As expected, the AvianPr NEP did not lead to a comparable increase of the AvianPr polymerase activity. 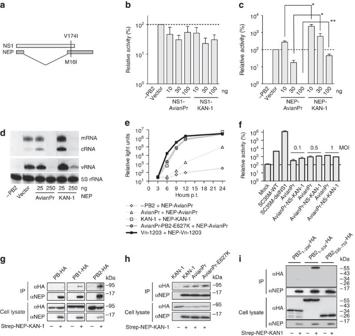Figure 5: Influence of NS segment-encoded proteins on polymerase activity. (a) Cartoon depicting the amino-acid mutations in NS1 and NEP of KAN-1 caused by a single nucleotide mutation in the KAN-1 NS segment. (b) Reporter activities after reconstitution of the AvianPr polymerase in HEK293 T cells and co-transfection of the indicated amounts of NS1-AvianPr, or NS1-KAN-1 encoding plasmids. Vector, empty plasmid. (c) Reporter activities after reconstitution of the AvianPr polymerase and co-transfection of the indicated amounts of NEP-AvianPr, or NEP-KAN-1 encoding plasmids. Student'st-test was performed to determine theP-value. *P<0.05, **P<0.01. Vector, empty plasmid. (d) Determination of the mRNA, cRNA and vRNA levels by primer extension analysis after reconstitution of the AvianPr polymerase in HEK293T cells and co-transfection of either empty plasmid (Vector), NEP-AvianPr or NEP-KAN-1 using primers specific for segment 6. Determination of the 5sRNA levels served as an internal loading control. (e) Time course of reporter activities of AvianPr, KAN-1 and Vn-1203 polymerases in HEK293T cells after co-transfection of 10 ng of the indicated NEP-expressing plasmids. (f) Interferon induction in infected cells. Mouse 3T3 cells stably transfected with a plasmid coding for firefly luciferase under the control of the interferon β-promoter were infected with AvianPr or AvianPr harbouring the NS-segment of KAN-1 (AvianPr-NS-KAN-1) at the indicated MOI. Mock infection or infection with either SC35M-WT or SC35M-delNS1 at a MOI of 0.5 known to induce β-interferon served as internal controls. Luciferase activity was determined after 16 h post infection. (g) Complex formation of NEP with either PB1, PA or PB2. Human 293T cells were transiently transfected with Strep-tagged KAN-1 NEP and the indicated HA-tagged polymerase subunits and subjected to co-immunoprecipitations (IP). Precipitated polymerase subunits were identified by western blot analysis, using specific antibodies against the HA- and the Strep-tag. (h) Binding of Strep-tagged KAN-1 NEP to the indicated PB2 variants and (i) to PB2 truncation mutants. Figure 5: Influence of NS segment-encoded proteins on polymerase activity. ( a ) Cartoon depicting the amino-acid mutations in NS1 and NEP of KAN-1 caused by a single nucleotide mutation in the KAN-1 NS segment. ( b ) Reporter activities after reconstitution of the AvianPr polymerase in HEK293 T cells and co-transfection of the indicated amounts of NS1-AvianPr, or NS1-KAN-1 encoding plasmids. Vector, empty plasmid. ( c ) Reporter activities after reconstitution of the AvianPr polymerase and co-transfection of the indicated amounts of NEP-AvianPr, or NEP-KAN-1 encoding plasmids. Student's t -test was performed to determine the P -value. * P <0.05, ** P <0.01. Vector, empty plasmid. ( d ) Determination of the mRNA, cRNA and vRNA levels by primer extension analysis after reconstitution of the AvianPr polymerase in HEK293T cells and co-transfection of either empty plasmid (Vector), NEP-AvianPr or NEP-KAN-1 using primers specific for segment 6. Determination of the 5sRNA levels served as an internal loading control. ( e ) Time course of reporter activities of AvianPr, KAN-1 and Vn-1203 polymerases in HEK293T cells after co-transfection of 10 ng of the indicated NEP-expressing plasmids. ( f ) Interferon induction in infected cells. Mouse 3T3 cells stably transfected with a plasmid coding for firefly luciferase under the control of the interferon β-promoter were infected with AvianPr or AvianPr harbouring the NS-segment of KAN-1 (AvianPr-NS-KAN-1) at the indicated MOI. Mock infection or infection with either SC35M-WT or SC35M-delNS1 at a MOI of 0.5 known to induce β-interferon served as internal controls. Luciferase activity was determined after 16 h post infection. ( g ) Complex formation of NEP with either PB1, PA or PB2. Human 293T cells were transiently transfected with Strep-tagged KAN-1 NEP and the indicated HA-tagged polymerase subunits and subjected to co-immunoprecipitations (IP). Precipitated polymerase subunits were identified by western blot analysis, using specific antibodies against the HA- and the Strep-tag. ( h ) Binding of Strep-tagged KAN-1 NEP to the indicated PB2 variants and ( i ) to PB2 truncation mutants. Full size image Figure 7: Identification of adaptive mutations in NEP of other human isolates. 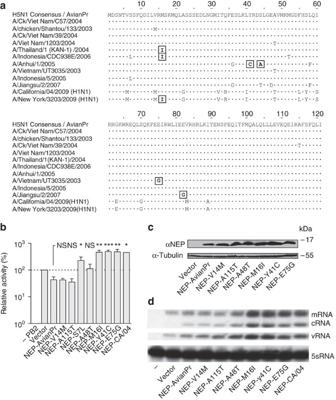Figure 7: Identification of adaptive mutations in NEP of other human isolates. (a) Sequence alignment of NEPs of human and avian H5N1 viruses as well as the NEP of the 2009 pandemic H1N1 virus to the H5N1 consensus sequence. Bold letters indicate amino acids exclusively found in human H5N1 isolates. (b) Reporter activities after reconstitution of the AvianPr polymerase in human HEK293T cells and co-transfection of 10 ng of expression plasmids coding for AvianPr NEP harbouring the indicated amino-acid substitution. Error bars indicate the s.e. of the mean of three independent experiments. Student'st-test was performed to determine theP-value. *P<0.05, **P<0.01, ***P<0.001, NS, not significant. NEP-M16I corresponds to NEP-KAN-1. (c) Western blot analysis of the NEP expression levels after transient transfection of HEK 293 T cells with equal amounts of expression plasmids (500 ng) encoding the indicated NEP variants. (d) Determination of the mRNA, cRNA and vRNA levels by primer extension analysis after reconstitution of the AvianPr polymerase in human HEK293 T cells and co-transfection of either empty plasmid (Vector) or AvianPr NEP harbouring the indicated amino-acid substitution using primers specific for segment 6. Determination of the 5sRNA levels served as an internal loading control. ( a ) Sequence alignment of NEPs of human and avian H5N1 viruses as well as the NEP of the 2009 pandemic H1N1 virus to the H5N1 consensus sequence. Bold letters indicate amino acids exclusively found in human H5N1 isolates. ( b ) Reporter activities after reconstitution of the AvianPr polymerase in human HEK293T cells and co-transfection of 10 ng of expression plasmids coding for AvianPr NEP harbouring the indicated amino-acid substitution. Error bars indicate the s.e. of the mean of three independent experiments. Student's t -test was performed to determine the P -value. * P <0.05, ** P <0.01, *** P <0.001, NS, not significant. NEP-M16I corresponds to NEP-KAN-1. ( c ) Western blot analysis of the NEP expression levels after transient transfection of HEK 293 T cells with equal amounts of expression plasmids (500 ng) encoding the indicated NEP variants. ( d ) Determination of the mRNA, cRNA and vRNA levels by primer extension analysis after reconstitution of the AvianPr polymerase in human HEK293 T cells and co-transfection of either empty plasmid (Vector) or AvianPr NEP harbouring the indicated amino-acid substitution using primers specific for segment 6. Determination of the 5sRNA levels served as an internal loading control. Full size image Because of the overlapping open-reading-frames coding for NS1 and NEP, we cannot formally exclude a contribution of the NS1 protein of KAN-1 in the adaptation process to human cells. However, we observed no difference in type I interferon induction between both strains after infection of a reporter cell line coding for firefly luciferase under the control of the interferon beta promoter with either AvianPr or AvianPr-NS-KAN-1 ( Fig. 5f ). We recently showed that NEP is associated with purified viral RNPs [20] . As NEP has been suggested to interact with the viral polymerase proteins in a yeast two-hybrid-screening [21] , and our results suggest that it might compensate for a defect in the viral polymerase, we tested whether these proteins physically associate using co-immunoprecipitation. KAN-1 NEP interacted with both PB1 and PB2, whereas no complex formation was detected with PA ( Fig. 5g ). Moreover, KAN-1 NEP associated with PB2 of KAN-1, AvianPr as well as Avian-Pr-E627K ( Fig. 5h ), suggesting that the protein interaction domain on PB2 is conserved in all three PB2 subunits. Using PB2 truncation mutants, we could further map the interaction of NEP to the amino-terminal part of PB2 comprising amino acids (aa) 1-534, containing the Cap-binding domain, but not to a shorter fragment (aa 1-299) or the C-terminal domain of PB2 (aa 535-759) ( Fig. 5i ). Together, these results indicate that the adaptive mutation M16I in the NEP protein of the KAN-1 virus enhances the capacity of NEP to stimulate viral polymerase activity, rendering NEP an essential cofactor in the adaptation process of the KAN-1 virus to a mammalian host. KAN-1 NS segment enhances RNA synthesis of AvianPr virus To investigate whether the RNA-synthesis-enhancing effect of the KAN-1 NEP is also relevant in the context of a viral infection, HEK293T cells were infected with the recombinant viruses AvianPr, KAN-1, AvianPr containing the KAN-1 NS segment (AvianPr-NS-KAN-1) and AvianPr with the polymerase harbouring the adaptive mutation E627K in the PB2 protein (AvianPr-PB2-E627K), respectively. To monitor early phases of viral RNA synthesis, total RNA from cells collected at 1, 2, 2.5 and 3 h post-infection (p.i.) were used for measuring the accumulation of vRNA, cRNA and viral mRNA by primer extension analysis. AvianPr failed to synthesize vRNAs to levels comparable to KAN-1 and AvianPr-PB2-E627K at any time point measured ( Fig. 6a,b ). However, introduction of the KAN-1 NS segment (AvianPr-NS-KAN-1) could rescue this defect and lead to enhanced synthesis of all three viral RNA species by the avian precursor polymerase ( Fig. 6a,b ). 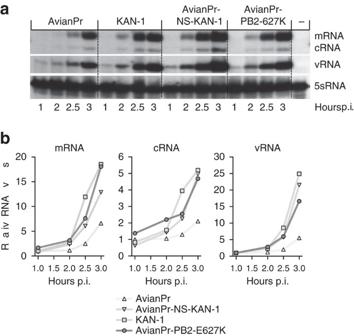Together, these results indicate that the non-adapted avian polymerase has a disadvantage to replicate efficiently in human cells in culture and that an adaptive mutation in either PB2 (E627K) or in NEP (M16I) can compensate for this defect. Figure 6: Accumulation of vRNAs during infection with recombinant viruses. (a) Human HEK293T cells were infected with an MOI of 5 with AvianPr, KAN-1, AvianPr-NS-KAN-1 and AvianPr-PB2-E627K. After the indicated time points post-infection (p.i.), cells were lysed and RNA levels were determined by primer extension analysis using primers specific for segment 6. Determination of the 5sRNA levels served as an internal loading control. −, primer extension analysis using uninfected cells.(b) Quantification of the radioactive signals shown in panel (a). Signals were normalized to 5sRNA level. Increase in mRNA and cRNA levels was normalized to the strain-specific vRNA levels at 1 h p.i. Figure 6: Accumulation of vRNAs during infection with recombinant viruses. ( a ) Human HEK293T cells were infected with an MOI of 5 with AvianPr, KAN-1, AvianPr-NS-KAN-1 and AvianPr-PB2-E627K. After the indicated time points post-infection (p.i. ), cells were lysed and RNA levels were determined by primer extension analysis using primers specific for segment 6. Determination of the 5sRNA levels served as an internal loading control. −, primer extension analysis using uninfected cells. ( b ) Quantification of the radioactive signals shown in panel ( a ). Signals were normalized to 5sRNA level. Increase in mRNA and cRNA levels was normalized to the strain-specific vRNA levels at 1 h p.i. Full size image NEPs of human PB2-E627 isolates enhance polymerase activity We could show that the adaptive mutation in the KAN-1 NEP protein increases its capacity to enhance the avian viral polymerase activity. This polymerase-enhancing activity is comparable to the effect mediated by the introduction of the PB2-E627K mutation into the AvianPr polymerase, suggesting that NEP may be an important pathogenicity factor for human influenza viruses that have retained the avian-like PB2-E627. We therefore investigated whether other H5N1 viruses encoding PB2-E627 contained adaptive mutations in NEP. Through sequence alignment, we identified additional avian and human clade 1 and clade 2 H5N1 isolates that contain PB2-E627 and differ by only a few amino acids from the AvianPr NEP, which resembles the consensus sequence of H5N1 viruses ( Fig. 7a ). Whereas the mutations V14M, A115T, A48T and S7L are found in avian and human isolates, the mutations Y41C and E75G are restricted to human isolates. The mutation S7L is mainly restricted to H5N1 strains from Indonesia and all 80 human isolates analysed of this subtype contain this mutation. These mutations were introduced into the AvianPr NEP protein to investigate their polymerase-enhancing capacity in the polymerase reconstitution assay. As the pandemic H1N1 virus also possesses PB2-E627 and is the dominant influenza A virus strain currently circulating in the human population, we also included the NEP of A/California/04/2009 (H1N1). In agreement with our assumption that only mutations in human-adapted strains lead to the enhanced NEP phenotype, the avian NEP variants harbouring the mutations V14M and A115T retrieved from the avian isolates did not lead to an increase in reporter activity ( Fig. 7b ). The mutation A48 T found in the human H5N1 isolate A/Viet Nam/1203/2004 (Vn-1203), which harbours PB2-K627, only weakly enhanced the reporter activity. In contrast, the human-derived mutations Y41C and E75G in avian NEP and also the pandemic H1N1 NEP protein were able to increase reporter gene activity to a similar extent as KAN-1 NEP ( Fig. 7b ). Western blot analysis confirmed comparable expression of these proteins ( Fig. 7c ). The increased enhancing activity of the pandemic H1N1 NEP and the NEP variants, containing the human-specific mutations Y41C and E75G, was further supported by primer extension analysis, which showed a strong increase in all three viral RNA species (vRNA, cRNA and mRNA) on co-expression ( Fig. 7d ). However, none of the NEP proteins encoding the avian-derived mutations V14M, A115T or A48T was able to raise vRNA levels to the same extent as KAN-1 NEP. Notably, the S7L mutation, found in avian and human H5N1 isolates, ( Fig. 7a ) also stimulated the AvianPr polymerase ( Fig. 7b ). Thus, the increased polymerase-enhancing phenotype of NEP can be achieved by many different amino-acid changes. Therefore, the utilization of NEP as a cofactor in the viral adaptation process to the human host is most likely not restricted to the KAN-1 virus, as it can also be observed for other human H5N1 isolates and the pandemic H1N1 strain containing the avian-like PB2-E627 signature. Infection of humans by avian influenza A viruses is a threat to the human population. Although viral replication of avian viruses, including pathogenic avian H5N1 strains, is impaired in human cells, incorporation of adaptive mutations enables the virus to overcome this defect. In this study, we characterized the supply of bona fide cRNA as the principal defect of avian polymerases in cultured human cells. Furthermore, we provide evidence that the polymerase of the human H5N1 isolate KAN-1, which encodes PB2-E627, is only partially able to compensate for this defect, and that the NEP of KAN-1 acquired an adaptive mutation (M16I) to stimulate the inefficient polymerase activity of this virus in human cells in culture. We further show that NEPs of circulating avian H5N1 viruses fail to compensate for the defect of avian viruses, whereas NEPs of H5N1 viruses isolated from humans encoding PB2-E627 contain adaptive mutations that enhance polymerase activity. Thus, we have identified an adaptive mutation of NEP as a potential alternative strategy for avian H5N1 viruses to cross the species barrier from birds to mammals. Our results suggest that the major defect of avian polymerases in human cells in culture is an impairment in vRNA replication. We observed that an avian polymerase (AvianPr), which normally produces only very low levels of viral mRNA, synthesized much higher amounts of mRNA when cRNA and vRNA were provided by an alternative polymerase ( Fig. 4b ), suggesting that the avian polymerase is specifically impaired in either cRNA or vRNA synthesis. Interestingly, both avian and human-like (AvianPr-PB2-E627K) polymerases synthesized cRNA to an equivalent extent ( Fig. 4e ). However, cRNA produced by AvianPr was unable to support robust vRNA synthesis in the presence of an active polymerase ( Fig. 4e , lane 5), whereas cRNA produced by AvianPr PB2-E627K supported robust vRNA synthesis ( Fig. 4e , lanes 4 and 6). On the basis of this finding, we speculate that avian polymerases do not have an impaired rate of overall RNA synthesis in human cells in vitro , but rather synthesize defective cRNPs, which are not bona fide templates for further RNA replication. This hypothesis is supported by our observation that AvianPr could efficiently synthesize vRNA, when provided with competent cRNPs ( Fig. 4e , lane 4), and by a previous report that showed that recombinant, purified polymerase is active in vitro regardless of the identity of PB2 residue 627 (ref. 22 ). Moreover, we observed reduced levels of cRNA after providing a competent polymerase compared with an incompetent polymerase ( Fig. 4e , compare lane 3 and 5 to lane 1). This suggests a decreased stability of cRNPs created by an avian influenza polymerase ( Fig. 8 ), as observed before for cRNPs at high temperature [23] . In summary, the well-known adaptive mutation PB2 E627K seems to confer the ability to correctly synthesize cRNPs to avian polymerases in human cells in culture. 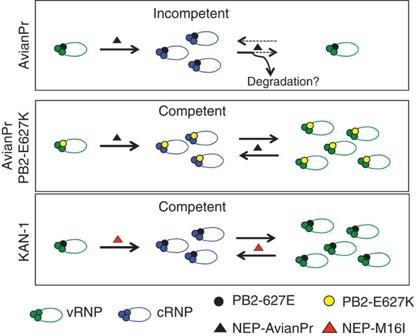Figure 8: Model of adaptive mutations contributing to the replication of avian H5N1 isolates in human cells. Our results suggest that cRNPs can be formed in human cells infected with AvianPr. Nevertheless, viral vRNP replication seems to be impaired, possible by premature degradation of cRNA. This defect in viral replication is not observed in cells infected with AvianPr PB2-E627K, indicating the single adaptive mutation E627K in PB2 is sufficient to overcome this defect. However, vRNPs are also efficiently generated in cells infected with human-derived H5N1 strains, such as KAN-1, lacking this human signature in PB2. In this case, the block in vRNP synthesis was overcome by a single adaptive mutation (M16I) in NEP of KAN-1 that increased the activity of this protein to enhance viral replication. Figure 8: Model of adaptive mutations contributing to the replication of avian H5N1 isolates in human cells. Our results suggest that cRNPs can be formed in human cells infected with AvianPr. Nevertheless, viral vRNP replication seems to be impaired, possible by premature degradation of cRNA. This defect in viral replication is not observed in cells infected with AvianPr PB2-E627K, indicating the single adaptive mutation E627K in PB2 is sufficient to overcome this defect. However, vRNPs are also efficiently generated in cells infected with human-derived H5N1 strains, such as KAN-1, lacking this human signature in PB2. In this case, the block in vRNP synthesis was overcome by a single adaptive mutation (M16I) in NEP of KAN-1 that increased the activity of this protein to enhance viral replication. Full size image Intriguingly, 71% of the human H5N1 virus isolates (127/179, Influenza virus research database) have not acquired the PB2-E627K mutation, likely reflecting an incomplete adaptation to human hosts. Nonetheless, many of these viruses are pathogenic, even fatal, in humans. Our results suggest that these viruses utilize NEP as a polymerase cofactor to elevate their low RNA replication capacity in humans ( Fig. 8 ). Adaptive mutations in NEP are required to efficiently stimulate avian and avian-like influenza polymerases. Interestingly, human H5N1 isolates that harbour the adaptive mutation E627K in PB2 do not contain adaptive mutations in NEP that enhance the polymerase activity to a similar degree as KAN-1 NEP ( Fig. 8 ). We therefore speculate that viruses such as Vn-1203, which possess highly active polymerases because of the PB2-E627K mutation, are not dependent on the additional replication-enhancing property of NEP ( Fig. 8 ). Interestingly, our data underscore that NEP interacts with the viral polymerase in human cells in culture, as we could show an association with PB1 and PB2. As both subunits have been implicated in promoter binding [24] , we speculate that association with NEP might also lead to a stabilization of cRNPs, thereby increasing the synthesis of vRNA transcripts, as suggested by others [25] . Although the KAN-1-specific adaptive mutation M16I is located within the nuclear export signal of NEP (aa 12–21) [26] , the replication-enhancing property of NEP is most likely independent of its export function [25] . In addition, treatment of human cultured cells with leptomycin B, an inhibitor of nuclear export, had no effect on the reporter-enhancing function of either KAN-1 NEP or AvianPr NEP (data not shown). Furthermore, other adaptive mutations found to enhance the polymerase activity (Y41C and E75G) are located outside the nuclear export signal motif. The latter mutation (E75G) is known to be involved in M1 binding [27] ; however, as M1 is not included in the polymerase reconstitution assay, it is unlikely to be relevant. Interestingly, we observed that the mutation S7L promoted the polymerase-enhancing activity of NEP. Sequence analysis revealed that this mutation is present in NEP of all avian and human H5N1 isolates from the Indonesian lineage. Correspondingly, 89% (80/90, Influenza virus research database) of the human isolates, originating from this lineage, have retained the avian like PB2-E627. We hypothesize that the acquisition of the mutation S7L in NEP is responsible for the high frequency of PB2-E627 in this lineage. Through an increased stimulatory effect of NEP on polymerase activity, this mutation possibly lowered the selective pressure on these viruses to obtain the PB2-E627K mutation in humans. Our identification of NEP as a pathogenicity factor that enables avian influenza viruses to perform efficient genome replication in human cells in culture, suggests that avian influenza viruses have developed multiple strategies to adapt to human hosts. The recognition of adaptive mutations in NEP might help to evaluate the potential risk of circulating avian viruses to the human population. Plasmid constructions pHW2000 vectors [28] were used for influenza A virus rescue. To obtain rescue plasmids containing segments that encode mutant genes, site-directed mutagenesis was performed. To create the pCAGGS expression plasmids encoding for mutant PB2, PB1 or PA, the required mutations were introduced by assembly PCR. The resulting PCR fragments were cloned into vectors expressing PB2 and PB1 with the restriction enzymes Not I and Xho I or PA using Not I and Nhe I. The NS1- and NEP-coding plasmids were cloned using the gene-specific forward and reverse primers for NS1 and NEP and cloned into pCAGGS vectors using Not I and Xho I. The pCAGGS expression plasmids encoding the respective C-terminally HA-tagged polymerase subunits (PA, PB1, PB2) or PB2 truncation mutants were generated by PCR and ligated into pCAGGS PA SC35M -HA vector [29] linearized with Xma I and Not I. The N-terminal Strep-tag [20] was cloned in pCAGGS-HA-NEP KAN−1 expression plasmid linearized with EcoR I and Not I. The corresponding cloning primers are specified in Supplementary Table S2 . Animal experiments All animal experiments were performed in compliance with the German animal protection law (TierSchG). The animal welfare committees of the University of Freiburg, as well as the local authorities approved all animal experiments. BALB/c mice were obtained from Janvier (Straßburg). Six-to-eight-week-old mice were anaesthetized with a mixture of ketamine (100 μg per gram body weight) and xylazine (5 μg per gram) administered intraperitoneally and inoculated intranasally with the indicated doses of viruses in 50 μl PBS containing 0.2% bovine serum albumin (BSA). Animals were killed, if severe symptoms developed, or body weight loss approached 25% of the initial value. Lung homogenates were prepared using the FastPrep24 system (MP Biomedicals). Briefly, after addition of 800 μl of PBS containing 0.2% BSA, lungs were subjected to two rounds of mechanical treatment for 10 s each at 6.5 m s −1 . Tissue debris was removed by low-speed centrifugation. The LD 50 values were calculated based on the infectious dose (PFU). Sequencing of viruses RNA purification was carried out using 800 μl of Trizol reagent and 200 μl of virus stock or lung homogenate. Purified RNA was reverse transcribed using the one-step RT–PCR kit (Roche) and PCR was performed with KAN-1 specific primers. Cells HEK293 T, 3T3 and MDCK II cells were grown in Dulbecco's modified Eagle's medium supplemented with 10% fetal calf serum, 2 mM L -glutamine and 1% penicillin/streptomycin. Chicken hepatocellular epithelial cell line (LMH) was grown in Dulbecco's modified Eagle's medium supplemented with 8% fetal calf serum 2% chicken serum, 2 mM L -glutamine and 1% penicillin/streptomycin. All cells were maintained at 37 °C and 5% CO 2 . Co-precipitation experiments were essentially carried out as described [30] using Strep-Tactin sepharose beads (IBA). Reconstitution of the influenza virus polymerase As described [31] , HEK293T cells seeded into a 12-well plate were transiently transfected with a plasmid mixture containing either influenza A virus PB1-, PB2-, PA- (50 ng each), NP-expression plasmids (200 ng), and a human polymerase I (Pol I) expression plasmid (25 ng) expressing an influenza virus-like RNA (vRNA-luciferase) coding for the reporter protein firefly luciferase to monitor viral polymerase activity. vRNA-luciferase was flanked by noncoding sequences of segment 8 of FluA. The transfection mixture also contained a plasmid constitutively expressing renilla luciferase (25 ng), which served to normalize variation in transfection efficiency. Reconstitution of the viral polymerase complex in avian cells was performed as above with the exception that avian LMH cells were transfected and the minigenome RNA was expressed under the control of a chicken Pol I promoter (kindly provided by Daniel Mayer). cRNA stabilization assay Confluent HEK293T cells in 6-well plates were transiently transfected with the pCAGGS expression plasmids coding for various polymerase subunits (250 ng) and NP (1,000 ng) using Lipofectamine 2000 (Invitrogen). Cells were subsequently infected with the indicated virus strains at a multiplicity of infection (MOI) of 5 in the presence of 100 μg of cycloheximide per ml, 16–18 h post-transfection. Primer extension analysis For determination of viral transcript levels of reconstituted polymerases, 6-well plates with confluent HEK293 T cells were transiently transfected with a plasmid mixture containing either FluA PB1-, PB2-, PA- (125 ng each), NP-expression plasmid (500 ng), and a polymerase I (Pol I)-expression plasmid (25 ng) expressing an influenza virus RNA coding for the segment 6 of FluA. 25 ng of empty vector or NEP expression plasmid was contransfected for experiments involving NEP. For determination of viral transcript levels in virus-infected HEK293T cells, cells were seeded in 6-well plates. Infection was carried out with infection media (Dulbecco's modified Eagle's medium supplemented with 0.2% BSA, 2 mM L -glutamine and 1% penicillin/streptomycin). For analysing primary viral transcription, cycloheximide (100 μg ml −1 ) was added to the infection media. After the indicated time point post-transfection or infection, cells were collected in Trizol and RNA was purified according to the manufacturer's protocol (Invitrogen). Primer extension analysis was performed using specific primers for the NA and PB2 segment (mRNA, cRNA and vRNA) and cellular ribosomal RNA (5sRNA). The primers used for primer extension analysis are specified in Supplementary Table S3 . Accession codes: The data have been deposited in the NCBI nucleotide core database under accession codes: FRB100000.1, CY111595 ; FRB100000.2, CY111596 ; FRB100000.3, CY111597 ; FRB100000.4, CY111598 ; FRB100000.5, CY111599 ; FRB100000.6, CY111600 ; FRB100000.7, CY111601 and FRB100000.8, CY111602 . How to cite this article: Mänz, B. et al . Adaptive mutations in NEP compensate for defective H5N1 RNA replication in cultured human cells. Nat. Commun. 3:802 doi: 10.1038/ncomms1804 (2012).